Cotton cytochrome P450 CYP82D regulates systemic cell death by modulating the octadecanoid pathway Plant oxylipins are derived from unsaturated fatty acids and play roles in plant growth and development as well as defence. Although recent studies have revealed that fatty acid metabolism is involved in systemic acquired resistance, the precise function of oxylipins in plant defence remains unknown. Here we report a cotton P450 gene SILENCE-INDUCED STEM NECROSIS ( SSN ), RNAi suppression of which causes a lesion mimic phenotype. SSN is also involved in jasmonate metabolism and the response to wounding. Fatty acid and oxylipin metabolite analysis showed that SSN overexpression causes hyperaccumulation of hydroxide and ketodiene fatty acids and reduced levels of 18:2 fatty acids, whereas silencing causes an imbalance in LOX (lipoxygenase) expression and excessive hydroperoxide fatty acid accumulation. We also show that an unknown oxylipin-derived factor is a putative mobile signal required for systemic cell death and hypothesize that SSN acts as a valve to regulate HR on pathogen infection. Plants are constantly challenged by a barrage of microbes, but only a small proportion succeed in causing disease due to the well-established immune system of plants. Plant innate immune systems comprise complex signalling networks that generally include two modes, pathogen-associated molecular pattern-triggered immunity (PTI) and effector-triggered immunity (ETI) [1] . PTI is induced when pathogen-associated molecular patterns, which are conserved molecules such as flagellin, are perceived by extracellular receptors, the so-called pattern recognition receptors, such as FLS2 (ref. 2 ). However, when PTI is suppressed by pathogen effectors, and they are transported into the cell, plants can re-establish pathogen resistance using other defence modes, such as ETI [3] . ETI is induced when the avirulence effectors produced by a pathogen are recognized by the corresponding plant resistance proteins [4] . ETI is often accompanied by the hypersensitive response (HR), which includes an oxidative burst, cell wall lignification, phytoalexin accumulation and induction of cell death of infected cells and the cells that surround them, to prevent the pathogen from spreading [5] , [6] . HR is a form of programmed cell death (PCD) in plants [7] , which results in necrotic lesion formation, sealing the pathogen in a tomb of dead cells. This process is also associated with salicylic acid (SA) accumulation, which induces the expression of PATHOGENESIS-RELATED ( PR ) genes and eventually establishes systemic acquired resistance (SAR) [8] , [9] . Interestingly, SAR can be triggered in tobacco wild-type (WT) scion grafted onto an SA-deficient rootstock [10] . SAR has also been found to be blocked when SA methyl transferase was silenced in primary infected leaves, and SAR was induced in upper untreated leaves when lower leaves were treated with MeSA. Therefore, MeSA is a proposed SAR signal in tobacco [11] . Jasmonate (JA) rapidly accumulates in the phloem and exudates as the leaves are challenged with the avirulent Pseudomonas syringae ; further, SAR can be mimicked by a foliar JA application and is abrogated in mutants with impaired JA synthesis or response [12] . In addition, the JA precursor 12-oxo-phytodienoic acid accumulates in SAR-induced potato plants [13] . Similarly, azelaic acid (AZA) is also derived from C18 fatty acids, and together with its induced protein AZELAIC ACID INDUCED 1 (AZI1) plays an important role in the systemic immune response [14] . Nevertheless, a recent study presents evidence that methyl salicylate and JA are non-essential for SAR in Arabidopsis , and AZA is a general marker for lipid peroxidation rather than a general immune signal [15] , [16] , [17] . Moreover, defective SAR in acyl carrier protein 4 ( acp4 ) mutant plants was also not due to impaired salicylate or JA-mediated plant hormone signalling pathways but was associated with impaired leaf cuticles [18] . Great efforts have been made to identify other SAR mobile signals, leading to the discovery of a lipid transfer protein, DIR 1 (ref. 19 ), which is a DIR1 -dependent G-3-P derivative [20] . The dehydroabietinal [21] and the non-protein amino acid pipecolic acid [22] are translocated signalling molecules. SFD1 and FAD7 function in the synthesis of plastid-synthesized lipids that are critical for SAR [17] , [23] . In addition, certain glycerolipid-dependent factors along with the DIR1 -encoded lipid transfer protein are essential for long-distance signalling in SAR [17] . Therefore, these data suggest that lipid metabolism is required to establish SAR. However, AZA or JA are oxylipins derived from octadecanoids (C18 fatty acid pathway) and are regarded as dispensable for SAR; thus, other lipids or oxylipins may be involved in SAR signal transmission but have not been discovered. Given the complexity of lipid metabolism, the nature of the mobile signal is still unclear. Although plant oxylipins are important to plant growth and defence, their biological properties are poorly understood. Only one such oxylipin, JA, has been studied to produce a relatively clear account of its anabolism and signal regulation pathway in recent years. Here we report identification of a gene SSN ( GhCYP82D) in cotton. Suppressing its expression causes a severe HR-like phenotype in cotton plants. Bioinformatics analysis shows that it belongs to the CYP82 family of cytochrome P450s. The function of SSN was analysed using genetic and metabolic approaches to reveal its role in lesion formation. SSN is specifically required for confining the production of a presumed mobile signal involved in systemic cell death by modulating a previously unknown biosynthetic pathway of oxylipins derived from octadecanoids in cotton. We propose that this pathway is involved in SAR signal formation, and these findings suggest a novel metabolic branch that might regulate the JA signalling pathway. Downregulation of GhCYP82D leads to lesion mimic phenotype In our previous work, we isolated an expressed sequence tag from a cDNA library in a screen for genes involved in cotton disease resistance following inoculation with Verticillium dahliae [24] . Three highly similar genes (above 94%) were identified in G. hirsutum genotype YZ1 each with 1,569-nucleotide open reading frames (ORFs) and putatively encoded proteins of 522 amino acids, with conserved domains that are characteristic of eukaryotic P450 proteins ( Supplementary Fig. 1 ). Sequence analysis revealed that they share 55% identity with PtCYP82D2 but only 48% with AtCYP82C2 ( Fig. 1a and Supplementary Fig. 1 ). Thus, GhCYP82D is a novel P450 subfamily in cotton. The expression profiles were determined using reverse transcriptase–PCR (RT–PCR) with primers for the conserved regions in this gene family. The results showed that they were specifically expressed in roots and cotyledons of seedlings ( Fig. 1b ), which is consistent with results from glucuronidase (GUS) activity detection using promoters from two family members ( Fig. 1c and Supplementary Fig. 2a,b ). The gene family is highly induced by multiple phytohormones ( Supplementary Fig. 3 ), including JA ( Fig. 1d and Supplementary Fig. 2c ), and is induced by V. dahliae infection in roots of the susceptible cotton line Ji11 compared with mock treatments ( Fig. 1e ). However, it is downregulated in the resistant cotton line 7124 ( Fig. 1f ). 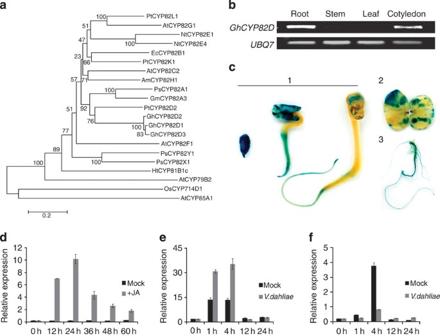Figure 1: Phylogenetic analysis of the CYP82 family and theSSNexpression pattern. (a) Protein phylogeny of the CYP82 family (P450 enzymes and proteins) fromGossypium hirsutum(Gh),Populus trichocarpa(Pt),Pisum sativum(Ps),Glycine max(Gm),Eschscholzia californica(Ec),Ammimajus(Am),Arabidopsis thaliana(At),Papaver somniferum(Ps),Nicotiana tabacum(Nt),Helianthus tuberosus(Ht) andOryza sativa(Os) plants. The neighbour-joining tree was constructed using the MEGA5 program (http://www.megasoftware.net/). (b) RT-PCR analysis ofGhCYP82Dexpression in different tissues. Total RNA was isolated from roots, stems, leaves and cotyledons of the WT cotton line YZ1. TheUBQ7gene was amplified as a control. (c)GhCYP82D1(SSN1) promoter::GUS fusion expression patterns in transgenic cotton. GUS staining was shown in germinating seeds (1), cotyledon (2) and root (3) of young seedlings. (d)GhCY82D(SSN) responses to JA treatments in cv. YZ1. The plants were pretreated with Hoagland’s solution; 25 μM JA was then added to the solution. (e) qRT–PCR showing theV. dahliae-inducedSSNexpression pattern in the susceptible cotton line Ji11. (f) qRT–PCR showing theV. dahliae-inducedSSNexpression pattern in the resistant cotton line 7124. The experiments (d–f) were repeated at least two times with similar results. The values are the means±s.d. for four technical replicates. The transcript levels of each gene were normalized toUBQ7. Figure 1: Phylogenetic analysis of the CYP82 family and the SSN expression pattern. ( a ) Protein phylogeny of the CYP82 family (P450 enzymes and proteins) from Gossypium hirsutum (Gh), Populus trichocarpa (Pt), Pisum sativum (Ps), Glycine max (Gm), Eschscholzia californica (Ec), Ammimajus (Am), Arabidopsis thaliana (At), Papaver somniferum (Ps), Nicotiana tabacum (Nt), Helianthus tuberosus (Ht) and Oryza sativa (Os) plants. The neighbour-joining tree was constructed using the MEGA5 program ( http://www.megasoftware.net/ ). ( b ) RT-PCR analysis of GhCYP82D expression in different tissues. Total RNA was isolated from roots, stems, leaves and cotyledons of the WT cotton line YZ1. The UBQ7 gene was amplified as a control. ( c ) GhCYP82D1 ( SSN1 ) promoter::GUS fusion expression patterns in transgenic cotton. GUS staining was shown in germinating seeds (1), cotyledon (2) and root (3) of young seedlings. ( d ) GhCY82D ( SSN ) responses to JA treatments in cv. YZ1. The plants were pretreated with Hoagland’s solution; 25 μM JA was then added to the solution. ( e ) qRT–PCR showing the V. dahliae -induced SSN expression pattern in the susceptible cotton line Ji11. ( f ) qRT–PCR showing the V. dahliae -induced SSN expression pattern in the resistant cotton line 7124. The experiments ( d – f ) were repeated at least two times with similar results. The values are the means±s.d. for four technical replicates. The transcript levels of each gene were normalized to UBQ7 . Full size image To explore the role of this P450 subfamily in cotton, we knocked down the expression of the gene family using RNA interference (RNAi) technology for the conserved regions. We also overexpressed the genes of this subfamily using the 35S promoter in transgenic cotton plants ( Supplementary Fig. 4 ). Most GhCYP82D RNAi seedlings showed lesion mimics on the stems and most died ( Fig. 2a and Supplementary Fig. 5a,b ), consistent with the level of gene downregulation ( Supplementary Fig. 5c ). The gene family was named SILENCING-INDUCED STEM NECROSIS ( SSN ), and the three members GhCYP82D1 , GhCYP82D2 and GhCYP82D3 were named SSN1 , SSN2 and SSN3 , respectively. No obvious phenotypic differences were observed between the SSN1 -, SSN2 -overexpressing and WT seedlings. A small number of GhCYP82D RNAi seedlings ( SSN -RNAi) survived showing the lesion mimic phenotype on the boll shell, bract and junction between the petiole and leaf in field-grown plants ( Fig. 2a and Supplementary Fig. 6a,b ). More serious necrosis was observed on the cotyledons when the SSN -RNAi-transgenic offspring were aseptically germinated in vitro ; the cotyledons fell approximately 9 days after germination ( Fig. 2b and Supplementary Fig. 7a,b ). The lesion mimic reappeared on the stems and cotyledons ( Fig. 2b and Supplementary Fig. 7c,d ), co-segregating with the downregulation of SSN ( Fig. 2c ). SSN -RNAi shoots were rescued by grafting to WT stems to obtain seeds. The transgenic offspring (lines Ri15 and Ri28) showed a strong necrosis phenotype, but the phenotype was inconspicuous for Ri54 ( Supplementary Fig. 6c ), linked to less SSN downregulation ( Supplementary Fig. 8a ). Low-copy-number insertions of SSN -RNAi, SSN1 -overexpression (OE1) and SSN2 -overexpression (OE2) plants were examined through western blotting ( Fig. 2d and Supplementary Fig. 8b ), which confirmed the downregulation and upregulation, respectively. 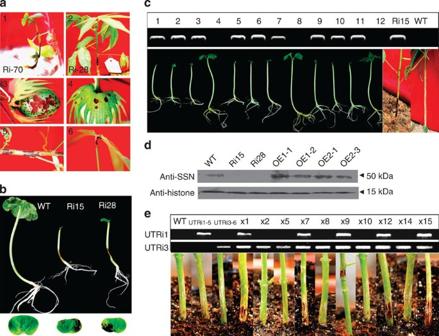Figure 2: Morphological features ofGhCYP82D(SSN)-RNAi plants grown in soil. (a) The lesion phenotype of RNAi transformants, showingSSN-RNAiin vitroplants (1), T0 plants in field to show lesions on the stem (2), boll shell (3), bract (4), branch (5) and junction with the petiole (6). (b) The lesion phenotype on stems and cotyledons ofSSN-RNAi T1 plants grown for 9 daysin vitro. (c) The cotyledons abscised from approximately 3/4 of the plants cultured for 9 daysin vitroamong the T1 segregations of theSSN-RNAi line Ri15. (d) Western blotting revealed different expression levels among the transgenic and WT plants leaves. Antibodies were prepared using the same SSN1 and SSN2 protein amino acid sequences as the probes; anti-histone was used as a control. Ri:SSN-RNAi plants; OE1:SSN1-overexpression plants; OE2:SSN2-overexpression plants. (e) The F1 plants were derived from a cross between homozygous UTRi3 (SSN3)-silenced plant and a heterozygous UTRi1 (SSN1)-silenced plant; one gene-specific primer (from 3′-UTR ofSSN1or 3′-UTR ofSSN3) and one vector primer (from the 35S promoter) were used to amplify the transgene in F1 plants, plants with both UTRi1 and UTRi3 amplified bands showed a lesion phenotype on the stems. Figure 2: Morphological features of GhCYP82D ( SSN )-RNAi plants grown in soil. ( a ) The lesion phenotype of RNAi transformants, showing SSN- RNAi in vitro plants (1), T0 plants in field to show lesions on the stem (2), boll shell (3), bract (4), branch (5) and junction with the petiole (6). ( b ) The lesion phenotype on stems and cotyledons of SSN -RNAi T1 plants grown for 9 days in vitro . ( c ) The cotyledons abscised from approximately 3/4 of the plants cultured for 9 days in vitro among the T1 segregations of the SSN -RNAi line Ri15. ( d ) Western blotting revealed different expression levels among the transgenic and WT plants leaves. Antibodies were prepared using the same SSN1 and SSN2 protein amino acid sequences as the probes; anti-histone was used as a control. Ri: SSN -RNAi plants; OE1: SSN1 -overexpression plants; OE2: SSN2 -overexpression plants. ( e ) The F1 plants were derived from a cross between homozygous UTRi3 ( SSN3 )-silenced plant and a heterozygous UTRi1 ( SSN1 )-silenced plant; one gene-specific primer (from 3′-UTR of SSN1 or 3′-UTR of SSN3 ) and one vector primer (from the 35S promoter) were used to amplify the transgene in F1 plants, plants with both UTRi1 and UTRi3 amplified bands showed a lesion phenotype on the stems. Full size image The HR-like phenotype is independent of SA synthesis To further explore the functional redundancy between the three members of the SSN family, RNAi-transgenic plants for the three members with specific 3′-UTR regions were generated and characterized by Southern blotting and quantitative RT-PCR (qRT-PCR; Supplementary Figs 4 and 8c–h ). Interestingly, the expression compensation was observed in the single-gene-silenced plants between any two members ( Supplementary Fig. 8c,e,h ). We did not observe any difference in growth between the single-gene-silenced and WT plants. Crossing was employed using different specific 3′-UTR silenced lines to examine the functional redundancy among the gene members. The results showed that silencing any two members of the SSN family could induce the lesion phenotype, as verified through an RNAi-segment analysis ( Fig. 2e and Supplementary Fig. 9 ). These results suggest that SSN members may have functional redundancy. A lesion phenotype is typically associated with cell death during HR to pathogens. HR always triggers the rapid production of reactive oxygen species and induces numerous PR genes [25] , [26] and is typically accompanied by SA accumulation [27] . To evaluate whether the lesion mimic in SSN -RNAi plants is due to HR-like cell death, the PR genes that are tightly correlated with the HR and H 2 O 2 level were analysed. The results show that many PR genes, including the commonly regarded marker genes PR1 and PR5 , were significantly upregulated in the SSN -RNAi stem. Further, CATALASE ( CAT ) was upregulated, and excess levels of H 2 O 2 were detected in the SSN -RNAi stem ( Fig. 3a ), which suggests that silencing SSN constitutively activates the HR in cotton seedlings. However, NPR1 expression was not influenced by SSN silencing in cotton seedlings. Moreover, the genes involved in SA biosynthesis, such as ICS1 , EDS1 and PAD4 , showed similar expression pattern to NPR1 , and we did not observe differences in SA levels between WT and SSN -RNAi seedling stems ( Fig. 3a ). In addition, PR1 upregulation was detected through RNA-gel blotting in different silenced lines ( Fig. 3b ), and excessive levels of H 2 O 2 shown by 3, 3′-diaminobenzidine (DAB) and 2′,7′-DCFDA staining were detected in the SSN-RNAi cotyledons and stems, further followed by necrosis and collapse of vascular bundle cells ( Fig. 3c , Supplementary Fig. 10 ). To investigate the involvement of SSN in the cotton response to V. dahliae , seedlings were inoculated with the V. dahliae strain ‘V991’. Compared with WT, resistance to V. dahliae was improved in SSN -RNAi but attenuated in OE seedlings ( Fig. 3d ). 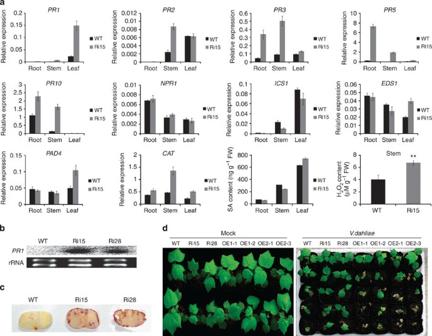Figure 3: Constitutively activated defence response inSSN-RNAi plants and disease resistance symptoms onV. dahliaeinfection. (a) The transcript levels ofPRgenes and SA biosynthesis genes and the H2O2levels in WT and Ri15 at the 10-day-old seedling before the lesion appeared on the plants. The SA levels of different tissues are from 3-week-old seedlings. The values are the means±s.d. for three biological replicates (**P<0.01, Student’st-test). (b) ThePR1gene expression level was determined using an RNA-gel blot analysis for leaves from 3-week-old seedlings. (c) H2O2accumulation at the site of lesion formation inSSN-RNAi cotyledons was visualized through DAB staining. (d) Disease symptoms among the WT,SSN-RNAi and OE lines after inoculation with theV. dahliaestrain ‘V991’. Three-week-old seedlings were root-wounded and dip-inoculated withV. dahliaebefore transplanted to soil. The photos were taken 12 days after inoculation. The experiments were repeated three times with similar results. Shown are representative symptoms of disease (at least 20 plants of each line). Figure 3: Constitutively activated defence response in SSN -RNAi plants and disease resistance symptoms on V. dahliae infection. ( a ) The transcript levels of PR genes and SA biosynthesis genes and the H 2 O 2 levels in WT and Ri15 at the 10-day-old seedling before the lesion appeared on the plants. The SA levels of different tissues are from 3-week-old seedlings. The values are the means±s.d. for three biological replicates (** P <0.01, Student’s t -test). ( b ) The PR1 gene expression level was determined using an RNA-gel blot analysis for leaves from 3-week-old seedlings. ( c ) H 2 O 2 accumulation at the site of lesion formation in SSN -RNAi cotyledons was visualized through DAB staining. ( d ) Disease symptoms among the WT, SSN -RNAi and OE lines after inoculation with the V. dahliae strain ‘V991’. Three-week-old seedlings were root-wounded and dip-inoculated with V. dahliae before transplanted to soil. The photos were taken 12 days after inoculation. The experiments were repeated three times with similar results. Shown are representative symptoms of disease (at least 20 plants of each line). Full size image These data suggest that SSN -RNAi seedlings exhibit a constitutively activated HR-like cell death phenotype, but this is independent of SA synthesis. SSN confers disease resistance by regulating JA anabolism To determine the function of SSN in the cotton immunity system, Illumina sequencing was employed to identify genes that were differentially expressed in roots between the SSN -RNAi (Ri15) and WT seedlings. We isolated 184 genes with different expression patterns between the two lines (RPKM>15 and the absolute value of log2 ratio >1 based on the false discovery rate (FDR) <0.001, Supplementary Table 1 ). Of these, 32 genes did not have corresponding homologous genes in Arabidopsis , and annotations for approximately 40 homologues in Arabidopsis are unknown. Approximately one-sixth of the remaining 112 genes have been shown to directly participate in JA and SA signalling pathways. Interestingly, all the genes involved in JA biosynthesis, such as LOX2 , AOS and AOC4 , and the signalling pathway, such as MYC2-like , JAZ1 , JAZ3 and JAZ10 , were upregulated in SSN -RNAi. However, the WRKY transcription factors involved in the SA signalling pathway, such as WRKY40 , WRKY50 , WRKY51 and WRKY70 , were downregulated in SSN -RNAi seedlings ( Table 1 and Supplementary Table 1 ). Certain genes were verified through qRT-PCR, and the results were consistent with the Illumina sequencing ( Supplementary Fig. 11a ). Silencing SSN in cotton upregulated genes related to JA biosynthesis, while the overexpression of SSN downregulated the expression level of genes involved in JA biosynthesis and decreased JA levels in leaves and stems ( Fig. 4a ). Table 1 Identification by Illumina sequencing of genes differentially expressed in WT and Ri15. 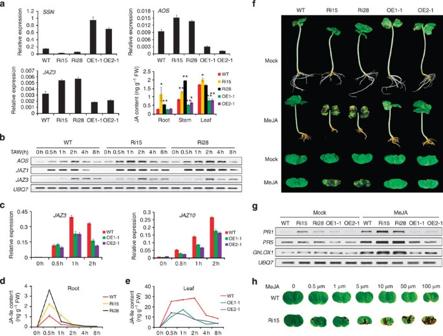Figure 4: SSN regulates the JA synthesis and signal transduction pathways. (a) Selected JA synthesis and signal transduction pathway genes from the RNA-Seq data were verified through qRT-PCR. RNA was extracted from roots of 6-day-old seedlings. Error bars indicate s.d. from four technical replicates. The JA levels were constitutively enhanced in 3-week-oldSSN-RNAi seedlings. The values are the means±s.d. for three biological replicates. The asterisks indicate statistically significant differences between the transgenic and WT plants (*P<0.05, **P<0.01, Student’st-test). (b) Time course forAOSandJAZmRNA accumulation analysed using RT–PCR in wounded roots of WT andSSN-RNAi. The total RNA was isolated from wounded roots of 3-week-old WT andSSN-RNAi plants. The cottonUBQ7gene was amplified as a control. TAW, time after wounding. (c) qRT–PCR amplification ofJAZgenes after wound treatment. Total RNA was extracted from 4-week-old WT and OE plants. Error bars indicate s.d. from four technical replicates. (d,e) Kinetics of wound-induced JA-Ile levels in roots and leaves. The values are the means±s.d. for three biological replicates. (f) Morphological phenotype shows that WT and transgenic seedlings grown for 5 days on media containing MeJA (5 μM) are sensitive to JA-induced growth inhibition.SSN-RNAi plants show more sensitivity to JA-mediated growth inhibition and exhibited accelerated and aggravated HR-like necrosis. (g) RT–PCR analysis of marker genes associated with HR in transgenic seedling cotyledons grown for 2 days on MeJA (5 μM) media. The cottonUBQ7gene was amplified as a control. (h) Photographs of WT and the Ri15 line grown for 4 days on media containing different MeJA concentrations. Full size table Figure 4: SSN regulates the JA synthesis and signal transduction pathways. ( a ) Selected JA synthesis and signal transduction pathway genes from the RNA-Seq data were verified through qRT-PCR. RNA was extracted from roots of 6-day-old seedlings. Error bars indicate s.d. from four technical replicates. The JA levels were constitutively enhanced in 3-week-old SSN -RNAi seedlings. The values are the means±s.d. for three biological replicates. The asterisks indicate statistically significant differences between the transgenic and WT plants (* P <0.05, ** P <0.01, Student’s t -test). ( b ) Time course for AOS and JAZ mRNA accumulation analysed using RT–PCR in wounded roots of WT and SSN -RNAi. The total RNA was isolated from wounded roots of 3-week-old WT and SSN -RNAi plants. The cotton UBQ7 gene was amplified as a control. TAW, time after wounding. ( c ) qRT–PCR amplification of JAZ genes after wound treatment. Total RNA was extracted from 4-week-old WT and OE plants. Error bars indicate s.d. from four technical replicates. ( d , e ) Kinetics of wound-induced JA-Ile levels in roots and leaves. The values are the means±s.d. for three biological replicates. ( f ) Morphological phenotype shows that WT and transgenic seedlings grown for 5 days on media containing MeJA (5 μM) are sensitive to JA-induced growth inhibition. SSN -RNAi plants show more sensitivity to JA-mediated growth inhibition and exhibited accelerated and aggravated HR-like necrosis. ( g ) RT–PCR analysis of marker genes associated with HR in transgenic seedling cotyledons grown for 2 days on MeJA (5 μM) media. The cotton UBQ7 gene was amplified as a control. ( h ) Photographs of WT and the Ri15 line grown for 4 days on media containing different MeJA concentrations. Full size image JA plays a role in the plant wound response. The expression patterns for genes involved in the JA signal pathway were examined in seedlings after experimental wounding. The results show that AOS , JAZ1 and JAZ3 expression levels were more rapidly induced in SSN -RNAi than WT seedlings ( Fig. 4b ). However, JAZ3 and JAZ10 transcripts were apparently attenuated in OE lines after a wound treatment compared with WT seedlings ( Fig. 4c ). In addition, we measured the jasmonoyl- L -isoleucine (JA-Ile) levels, which is the activated form of JA. Consistent with the kinetics of gene expression, SSN -RNAi plants hyperaccumulated JA-Ile levels compared with WT plants at the 0- to 2-h time points after wounding ( Fig. 4d ). In contrast to the elevated JA-Ile levels in silenced plants, lower JA-Ile levels in the OE lines correlated with lower gene expression ( Fig. 4e ). This shows that JA biosynthesis was partially blocked by the SSN overexpression, and wound signal transduction was also weakened due to the reduced JA. To further determine whether SSN are P450 enzymes that are directly involved in the catalytic effect on JA, 5-μM MeJA was applied into the MS medium. The seedling root growth for the WT and OE seedlings did not differ. However, SSN -RNAi seedlings showed an increased response to the exogenous MeJA treatment, with clear root growth inhibition and hypocotyl elongation retardation associated with constitutively active JA synthesis ( Fig. 4f ). Similar results were obtained using 1-μM MeJA ( Supplementary Fig. 11b ). Moreover, exogenous MeJA treatment accelerated and aggravated HR-like necrosis on SSN -RNAi cotyledons ( Fig. 4f ). Further, the expression levels of marker genes associated with HR were upregulated more intensively for SSN -RNAi during the MeJA treatment compared with the WT. In contrast, the expression levels for these genes were attenuated in the OE seedlings ( Fig. 4g ). In addition, with the increase in MeJA concentration, SSN -RNAi cotyledon necrosis was more dramatic and spread more rapidly, but necrosis was not observed in WT ( Fig. 4h ). AZA, which is the metabolite from the oxylipin pathway and was identified as a mobile signal of SAR [14] , upregulated the expression of SSN and suppressed the expression of AZI1 which was required for SAR in the roots of cotton seedlings ( Supplementary Fig. 12a,b ). HR-like necrosis in SSN -RNAi was accelerated and aggravated by an exogenous AZA treatment ( Supplementary Fig. 12c ). With increasing AZA concentrations, necrosis was observed in the cotyledon and the SSN -RNAi seedlings died rapidly ( Supplementary Fig. 12d ). In addition to the 13-LOX gene ( LOX2 ), which is involved in JA biosynthesis [28] , two other 9-LOX genes ( LOX1 and LOX5 ; Supplementary Fig. 11a ) in the JA biosynthesis branch [29] were found in the RNA-seq data, but the precise metabolic pathways are unclear [30] . However, previous result showed that GhLOX1 was involved in the cotton HR [31] . SSN is involved in fatty acid and oxylipin metabolism Previous studies have shown that constitutively activated JA biosynthesis and signalling do not induce lesion mimics [32] ; however, certain oxylipins mediate reactive oxygen species production and cell death in plants [33] , [34] . The results above suggest that SSN may be involved in oxylipin metabolism. We characterized the expression profiles for genes involved in the octadecanoid pathway in transgenic plants ( Fig. 5a and Supplementary Fig. 13a ). The results show that the expression levels of genes involved in 18:2 fatty acid metabolism, such as FAD7 , FAD8 , GhLOX1 , LOX2 , a-DOX1 and a-DOX2 were significantly inhibited in OE seedling roots compared with WT and SSN -RNAi ( Fig. 5a ). We applied individually oleic acid (OA, 18:1), linoleic acid (LA, 18:2) and α-linolenic acid (ALA, 18:3) to WT seedlings, and examined the SSN expression pattern. SSN expression patterns were the same as GhLOX1 , which uses LA and ALA as substrates ( Fig. 5c and Supplementary Fig. 13b ). Nevertheless, OA could induce GhLOX1 expression, but not SSN expression ( Fig. 5b ). Further, SSN was upregulated in cotton seedling roots when GhLOX1 and LOX2 were silenced, individually, through virus-induced gene silencing ( Fig. 5d,e ). 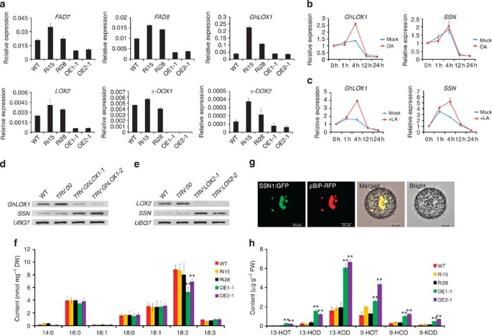Figure 5: SSN significantly modulates the metabolism of oxylipins derived from the octadecanoid pathway. (a) The key genes selected from 18:2 fatty acid metabolism pathway showed different expression patterns in theSSN-RNAi and OE lines. RNA was extracted from roots of 6-day-old seedlings. Error bars indicate s.d. from four technical replicates. The transcript levels of each gene were normalized toUBQ7. (b,c) TheGhLOX1andSSNexpression patterns responded to the oleic acid (OA) and linoleic acid (LA) treatments in cotton cotyledon, as demonstrated using qRT–PCR. RNA was extracted from seedlings at different intervals after an OA (10 mM) or LA (10 mM) application. Error bars indicate s.d. from four technical replicates. (d) RT–PCR analysis ofSSNexpression levels in WT,TRV:00andTRV:GhLOX1leaves. (e) RT-PCR analysis of the expression levels ofSSNin WT,TRV:00andTRV:LOX2leaves. (f) Fatty acid composition in the WT and transgenic line cotyledons. The values are the means±s.d. for four biological replicates. The asterisks indicate statistically significant differences between the transgenic and WT plants (**P<0.01, Student’st-test). (g) Subcellular localization of theSSN1gene product. From left to right: the protoplast showed green fluorescent signal at 488 nm; the same protoplast showed red fluorescent signal at 561 nm; image of the green and red signals; bright-field image. The data represent transformed protoplasts. The green and red fluorescent signals were examined 24 h after transformation. At least three independent transformation experiments were performed using the two constructs. Scale bars, 20 μm. (h) Major oxylipin compositions for 9/13 hydroxy-FAs and keto-FAs in the WT and transgenic line leaves. 9- or 13-HOT: 9- or 13-hydroxy octadecatrienoic acid; 9- or 13-HOD; 9- or 13-hydroxy octadecadienoic acid; 9- or 13-KOD; 9- or 13-keto octadecadienoic acid. The values are the means±s.d. for three biological replicates. The asterisks indicate statistically significant differences between the transgenic and WT plants (*P<0.05, **P<0.01, Studentst-test). Figure 5: SSN significantly modulates the metabolism of oxylipins derived from the octadecanoid pathway. ( a ) The key genes selected from 18:2 fatty acid metabolism pathway showed different expression patterns in the SSN -RNAi and OE lines. RNA was extracted from roots of 6-day-old seedlings. Error bars indicate s.d. from four technical replicates. The transcript levels of each gene were normalized to UBQ7 . ( b , c ) The GhLOX1 and SSN expression patterns responded to the oleic acid (OA) and linoleic acid (LA) treatments in cotton cotyledon, as demonstrated using qRT–PCR. RNA was extracted from seedlings at different intervals after an OA (10 mM) or LA (10 mM) application. Error bars indicate s.d. from four technical replicates. ( d ) RT–PCR analysis of SSN expression levels in WT, TRV:00 and TRV:GhLOX1 leaves. ( e ) RT-PCR analysis of the expression levels of SSN in WT, TRV:00 and TRV:LOX2 leaves. ( f ) Fatty acid composition in the WT and transgenic line cotyledons. The values are the means±s.d. for four biological replicates. The asterisks indicate statistically significant differences between the transgenic and WT plants (** P <0.01, Student’s t -test). ( g ) Subcellular localization of the SSN1 gene product. From left to right: the protoplast showed green fluorescent signal at 488 nm; the same protoplast showed red fluorescent signal at 561 nm; image of the green and red signals; bright-field image. The data represent transformed protoplasts. The green and red fluorescent signals were examined 24 h after transformation. At least three independent transformation experiments were performed using the two constructs. Scale bars, 20 μm. ( h ) Major oxylipin compositions for 9/13 hydroxy-FAs and keto-FAs in the WT and transgenic line leaves. 9- or 13-HOT: 9- or 13-hydroxy octadecatrienoic acid; 9- or 13-HOD; 9- or 13-hydroxy octadecadienoic acid; 9- or 13-KOD; 9- or 13-keto octadecadienoic acid. The values are the means±s.d. for three biological replicates. The asterisks indicate statistically significant differences between the transgenic and WT plants (* P <0.05, ** P <0.01, Students t -test). Full size image To assess the metabolic differences between the SSN -RNAi and OE lines, fatty acid levels were determined. Interestingly, only LA levels were significantly reduced in the OE seedlings compared with WT and SSN -RNAi ( Fig. 5f ). Furthermore, SSN-green fluorescent protein fusion protein localization indicates that SSN1 is an endoplasmic reticulum-localized protein ( Fig. 5g ). Further, transmission electron microscopy analyses on WT and transgenic seedling cotyledons suggest that SSN expression may influence plasmid development ( Supplementary Fig. 13c ). The cotyledon oxylipins were also measured, and 9-HOD/T, 13-HOD/T and 9/13-KOD dramatically accumulated in the OE seedlings ( Fig. 5h ). These data indicate that SSN is involved in the octadecanoid pathway. HR-like phenotype is related to imbalance in LOX pathway LOX-dependent hydroperoxide fatty acid formation is necessary for hypersensitive cell death development in plants, such as cotton [31] , [35] , pepper [36] and tobacco [37] . Because OE seedlings accumulate more hydroxy and keto C18 fatty acids, SSN likely acts on C18 fatty acids and competes for substrates with LOXs. We therefore hypothesized that SSN might modulate fatty acids metabolism in a novel pathway that differs from the pathway LOXs are involved in, and SSN inhibition leads to free fatty acid accumulation, which enhances LOXs expression and results in lipid peroxidation. To investigate this hypothesis, cotyledons from seedlings after germination at different lesion mimic formation stages were harvested for gene expression and hydroperoxide fatty acid composition analyses ( Fig. 6a ). The results show that SSN silencing strengthens the other two oxylipin metabolism pathways by forming 9-HPOs from 9-LOX and 13-HPOs from 13-LOX. During cotyledon development, GhLOX1 expression was constitutively active and reached a maximum as the lesion was observable in cotyledons ( Fig. 6b ). Moreover, the levels of oxylipins, 9-HPOD/9-HPOT metabolized by GhLOX1 (9-LOX) and 13-HPOD/13-HPOT metabolized by LOX2 (13-LOX) accumulated dramatically during SSN -RNAi cotyledon development ( Fig. 6d ). Consequently, the genes involved in the JA biosynthesis pathway were constitutively activated, and the JA levels clearly increased in SSN -RNAi cotyledons ( Fig. 6c and Supplementary Fig. 14 ). 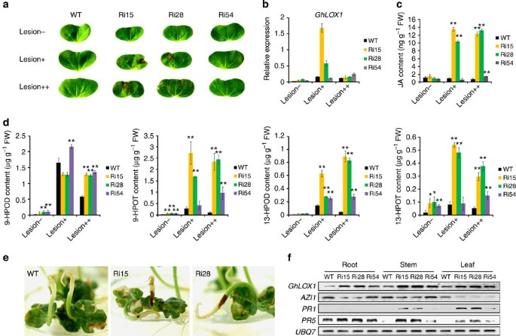Figure 6: The 9-LOX pathway plays an important role in systemic cell death. (a) Shown are different stages of lesion formation: 5-day-old seedlings before the lesion appears (lesion−), 7-day-old seedlings when the lesion appears (lesion+) and 8-day-old seedlings after the lesion forms (lesion++). (b) Transcript levels of the 9-LOX geneGhLOX1at the different lesion formation stages shown ina. Total RNA was extracted from cotyledon as shown inaand subjected to a qRT-PCR analysis. (c) JA levels stood for 13-LOX (LOX2) pathway activation in cotyledon tissue from the same set of plants used ina. (d) The products (9- or 13-HPOD/T) of the 9-LOX or 13-LOX enzymes in the cotyledon tissue froma. The values (b–d) are the means±s.d. of three biological replicates. The asterisks indicate statistically significant differences between the transgenic and WT plants (*P<0.05, **P<0.01, Student’st-test). (e) GerminatingSSN-RNAi seeds on the medium where the roots were not placed into medium manually also show a lesion phenotype on the stems. (f) TheGhLOX1,AZI1,PR1andPR5gene transcript levels in different tissues (root, stem and leaf) ofSSN-RNAi plants before the lesion phenotype appears. Total RNA extracted from different tissues of 3-week-old seedlings was subjected to RT–PCR analysis. Figure 6: The 9-LOX pathway plays an important role in systemic cell death. ( a ) Shown are different stages of lesion formation: 5-day-old seedlings before the lesion appears (lesion−), 7-day-old seedlings when the lesion appears (lesion+) and 8-day-old seedlings after the lesion forms (lesion++). ( b ) Transcript levels of the 9-LOX gene GhLOX1 at the different lesion formation stages shown in a . Total RNA was extracted from cotyledon as shown in a and subjected to a qRT-PCR analysis. ( c ) JA levels stood for 13-LOX ( LOX2 ) pathway activation in cotyledon tissue from the same set of plants used in a . ( d ) The products (9- or 13-HPOD/T) of the 9-LOX or 13-LOX enzymes in the cotyledon tissue from a . The values ( b – d ) are the means±s.d. of three biological replicates. The asterisks indicate statistically significant differences between the transgenic and WT plants (* P <0.05, ** P <0.01, Student’s t -test). ( e ) Germinating SSN -RNAi seeds on the medium where the roots were not placed into medium manually also show a lesion phenotype on the stems. ( f ) The GhLOX1 , AZI1 , PR1 and PR5 gene transcript levels in different tissues (root, stem and leaf) of SSN -RNAi plants before the lesion phenotype appears. Total RNA extracted from different tissues of 3-week-old seedlings was subjected to RT–PCR analysis. Full size image It is difficult to understand why the lesion could form on the stems, where the SSN gene expression was not detected, but the expression was rich in roots, where lesions were not observed. To investigate this, seeds were germinated in vitro without placing the roots into the medium manually, to allow the roots access to oxygen, but lesions were still not observed on the roots ( Fig. 6e ). We assume that a lipid-derived substance or signal in the roots may exist, and this signal could be transported to, and excessively accumulate in, the stems and this leads to lesion formation. To test this hypothesis, root, stem and leaf tissues were harvested from silenced and WT plants for biochemical analyses. The results show that GhLOX1 and PR5 transcripts were significantly upregulated in the stems and leaves compared with the SSN -RNAi seedling roots. In addition, high PR1 expression levels were only detected in SSN -RNAi leaves, and the AZI1 expression level was downregulated before lesion formation ( Fig. 6f ). We then performed a grafting study using WT and SSN -RNAi. SAR marker genes, such as PR1 and PR5 , were dramatically upregulated in leaves when the WT shoots were grafted onto stocks with SSN -RNAi as the rootstocks compared with the control, WT shoots grafted onto WT rootstocks. Further, the GhLOX1 expression pattern showed a similar trend to the PR genes, and the AZI1 expression level was downregulated in the heterografted WT:: SSN -RNAi leaves. However, we did not observe a significant difference in the leaf NPR1 and SSN expression levels after grafting ( Supplementary Fig. 15 ). Cytochrome P450s are one of the largest plant protein families, and are involved in a wide range of primary and secondary metabolic biosynthesis pathways. According to phylogenetic studies, P450s in the plant kingdom are divided into 10 separate clans in 61 families [38] . In this study, we isolated and characterized a novel P450 subfamily, CYP82D (SSN), in cotton. However, little information is available about the biochemical functions of the CYP82D subfamily in plants. Members of the CYP82 family ( Fig. 1a ) respond to stress in pea, tobacco and soybean [39] , [40] , [41] . Recent studies show that the CYP82 gene plays a role in Arabidopsis pathogen and herbivore resistance [42] , [43] , which led us to speculate that SSN may be involved in a specific area of secondary metabolism that is important for abiotic and biotic stress. Here we show that SSN -RNAi plants display spontaneous HR-like cell death with high PR gene expression. However, content analysis shows that the cell death phenotype is independent of a high level of endogenous SA, which is typically thought of as an essential condition for lesion mimic formation in many Arabidopsis mutants. We therefore speculate that cotton HR is regulated by a mechanism, which is independent of the SA pathway. SSN is highly expressed in cotyledons, and SSN silencing led to excessive JA accumulation, which implies that SSN may participate in lipid metabolism. Identifying SSN provides new insight into the function of a P450 subfamily, for which the physiological role in plants hitherto remains largely unknown. In addition, these data are helpful for discerning the relationship between the HR and JA or lipid metabolism, especially through the octadecanoid pathway. Generally, the cell death with lesion mimic phenotype was thought as a typical symptom of the HR in plant disease resistance. It is a suicide mechanism response to pathogen infection, similar to PCD in animals [44] . Previous studies show that animal and plant cells share a similar signal transduction pathway that triggers apoptosis and is derived from lipoxygenase activation [45] . Animal oxylipins have been associated with the inflammatory response and apoptotic pathway [46] . Therefore, elucidating the cellular processes that govern oxylipin homeostasis derived from lipoxygenase is essential for understanding the plant HR- and defence-related processes. Here we show that SSN regulates HR in cotton by modulating oxylipin metabolism. Metabolite analysis indicates that SSN defines a major pathway for lipid catabolism in the seedling stage. Given the JA-induced and wound-induced SSN expression, SSN activity may be involved in the JA pathway. The observed hydroperoxy fatty acid overproduction in SSN -RNAi cotyledons indicates that this pathway governs a negative regulatory mechanism, which effectively restrains uncontrollable hydroperoxide accumulation. This possibility is consistent with the time course for wound-induced JA-Ile derived from 13-hydroperoxy fatty acids, which shows greater accumulation in silenced plants but lower accumulation in OE plants on tissue damage. JA biosynthesis was partially blocked by SSN overexpression. Further, SSN co-expresses with the gene GhLOX1 , which is involved in LA and ALA metabolism as well as induced by LA and ALA treatment. Silencing SSN could induce LOX expression, and meanwhile, SSN expression was induced when the LOXs are silenced. As expected, significantly reduced levels of the fatty acid 18:2 were detected in overexpressing plants followed by over-accumulation of hydroxy and keto fatty acids. Our results support a hypothesis that SSN could act in a certain way for the metabolism of fatty acid-derived secondary metabolites by modulating JAs and fatty acid hydroxides synthesis. Grafting experiments are typically used to discern whether substances or signals are transferred from the root to shoots. Grafting the WT shoots to the SSN -RNAi rootstocks showed that certain substances or signals may be generated by the SSN -RNAi roots and transmitted to the WT shoots, which leads to an activated defence response. Moreover, when the seedlings were grown freely in vitro with oxygenated roots, the lesions only appeared on the stems, not the roots. This implies that there may be a mobile signal produced in the roots that triggers systemic cell death in the stems. SSN may be required to regulate the mobile signal generation and accumulation; seemingly, this signal is derived from the LOX pathway and positively regulates LOX expression. LOX-dependent hydroperoxide fatty acid formation is necessary for hypersensitive cell death development in tobacco [33] , [47] . GhLOX1 mediates cell death during the cotton HR when it interacts with Xcm ( Xanthomonas Campestris pv. Malvacearum ) [31] , [35] . The pepper 9-lipoxygenase gene CaLOX1 positively regulates defence responses and hypersensitive cell death [36] . Thus, GhLOX1 plays a central role as positive regulator of HR. Further, fatty acid hydroperoxides, LOX products, can induce PCD in tomato [48] and a recent study showed that oxylipin metabolism is a critical pathway that positively regulates PCD process during compatible interactions [37] . However, no oxylipins have been reported to induce HR as transferable elements or signal molecules. Our study suggests HPOD/HPOT may not only act as a substrate for either HPL or AOS to drive the GLV or JA pathway, but they or another unknown compound derived from them may also act as a long-distance mobile signal for systemic cell death. Moreover, they induced HR and PR gene expression. However, it is difficult to understand how the substance or signal was transferred. Recent work has shown that JA and AZA, which belong to this oxylipin pathway, may operate as the mobile signals [12] , [14] ; however, several studies disagree with those results [15] , [16] . Although the precise compounds have not been identified, more signal molecules have been documented, such as the lipid transfer protein DIR1 , a G3P-dependent signal, glycerolipid, cuticle and 12-oxo-phytodienoic acid [13] , [17] , [18] , [19] , [20] . Few studies have provided links between these putative signals. Our studies raise the hypothesis that an oxylipin-derived factor of C18 fatty acids is not only required for systemic cell death but also may partially affect the transmission of SAR signalling. Thus, JA or AZA may result from the SAR generation process, not form the basis for SAR signalling transmission. Furthermore, glycerol may promote lesion mimic formation and PR gene expression on silenced plant cotyledons ( Supplementary Fig. 16 ). Previous studies have shown that oxylipins occur not only in free form but can also be bound to phospholipids, glycolipids and neutral lipids [49] . On the basis of our results, we propose that suppressed SSN expression leads to an upset in the balance of oxylipin homeostasis, which in turn controls the ‘on/off’ signal for SAR. Traditionally, plants were thought to protect themselves against biotrophic and necrotrophic pathogens through distinct mechanisms, with the SA pathway generally effective against biotrophic or hemibiotrophic pathogens. The SSN -RNAi plants show resistance to V. dahliae , which is a hemibiotrophic pathogen that causes serious vascular disease in cotton on infection in underground root tissue [50] . However, the SA signalling pathway was suppressed by constitutively activated JA pathway in SSN -RNAi roots. This observation is explicable based on our studies. First, SSN was downregulated in the resistant cotton line but upregulated in the susceptible cotton line on V. dahliae infection. Although the specific mechanism of disease resistance has been unclear until now, SSN silencing in the susceptible cotton line YZ1 is the same as in resistance response of the downregulation process in resistant cotton line 7124. Second, we inoculated cotton seedlings by dipping the wound roots into a V. dahliae spore suspension, and greater JA-Ile accumulation was documented in wounded roots of SSN -RNAi plants ( Fig. 4d ). Further, recent research has shown that the JA pathway is important to V. dahliae infection [51] , [52] . Thus, we propose that JA, rather than SA, plays a key role in cotton V. dahliae resistance. Plant materials and growth conditions The cotton plants Gossypium barbadense cv. 7124, Gossypium hirsutum cv. Ji11 and Gossypium hirsutum cv. YZ1, as well as transgenic lines derived from YZ1 in these experiments, were cultivated in Wuhan, China under normal farming practices or grown in the greenhouse during the winter. The greenhouses were maintained at a temperature of 28–35/20–28 °C day/night. The roots, stems, cotyledons and leaves were collected from seedlings cultured in a growth chamber or in Hoagland’s solution. The collected materials were preserved at −80 °C until required for further analysis. Plant treatments For the JA/MeJA or AZA treatments using seedlings grown in Hoagland’s solution, 25 μM JA, 50 μM MeJA or 1 mM AZA (Sigma) was added to the Hoagland’s solution for the WT YZ1 plants (3 weeks), and the controls were added with ethanol to 0.01 or 0.2%. For the SA or ACC treatment, the cotton line YZ1 (3 weeks old) was grown in Hoagland’s solution, and 0.5 mM SA or 5 μM ACC (Sigma) was added; water was added to the controls. For the MeJA treatment in the medium, the WT and transgenic cotton lines were grown on a half-strength MS medium for 1.5 days and were then transferred to a mock treatment (0.01% ethanol) and media containing different concentrations of JA. For the AZA treatment on the medium, the WT and transgenic cotton lines were grown on a half-strength MS medium for 1.5 days; they were then transferred to a mock treatment (0.1% ethanol) and media containing the required AZA concentrations. For the glycerol treatment on the medium, the WT and transgenic cotton lines were grown on half-strength MS medium for 1.5 days; they were then transferred to a half-strength MS medium supplemented with or without 0.5% glycerol. For the FA treatment, FA stock solutions (200 mM) were prepared in 80% ethanol. Working solutions (10 mM) were prepared in deionized water with the surfactant SilwetL77 (0.02%). Mock solutions were prepared with ethanol (1%) and surfactant (0.02%) in deionized water. Cotyledons from the WT cotton line YZ1 (1 week old) were grown in a conical flask and sprayed with mock treatment or 10 mM various FAs (OA, LA and ALA), respectively. The tissues were then harvested at the indicated time intervals for RNA extraction. Wound treatment For silenced plants, the taproots of 3-week-old plants were grown in Hoagland’s solution and cut to lengths of ~1 cm using scissors. At various time points after wounding, the roots (four or five plants) were harvested, immediately frozen in liquid nitrogen and stored at −80 °C until they were used for RNA or JA extraction. For the overexpressing plants, fully expanded true leaves of 4-week-old plants were wounded to ~40% of the leaf area by crushing the leaf across the midrib using a haemostat. The leaves (four or five plants) were harvested as described above. Pathogen infection G. barbadense cv. 7124 and G. hirsutum cv. Ji11 seeds were grown in commercial sterilized soil for 3 weeks. The plants were inoculated with the V. dahliae strain V991, as described previously [24] . The plant roots were harvested for RNA extraction at 0, 1, 4, 12 and 24 h after inoculation. The control plants were treated with water and sampled at the same time points. Roots from five individual seedlings were collected for each treatment at each sampling time point. Roots from 3-week-old Hoagland’s solution-cultured WT and transgenic plant seedlings were separately wounded with scissors and dip-inoculated with the V. dahliae strain V991 to observe the disease symptoms. SSN cloning and sequence analysis Total RNA was extracted from cv. YZ1 or cv. 7124 roots using the guanidine thiocyanate method [53] . The first strand of cDNA was synthesized using the SuperScript III reverse transcriptase (Invitrogen, Carlsbad, CA, USA). The expressed sequence tag sequence was isolated from a suppression subtractive hybridization library of cotton line 7124 (ref. 24 ). The full-length sequence was obtained through 5′- and 3′-rapid amplification of the cDNA end (5′- and 3′-RACE) in accordance with the GeneRacer Kit user manual (Invitrogen) using cv. YZ1 cDNA as the PCR template. The ORF was predicted using ORF Finder ( http://www.ncbi.nlm.nih.gov/gorf/gorf.html ). Three genes with highly similar sequences were found during the sequencing process, which are referred to as GhCYP82D1 , GhCYP82D2 and GhCYP82D3 . The primer sequences are listed in Supplementary Table 2 . A sequence similarity analysis was performed using BOXSHADE software ( http://www.ch.embnet.org/software/BOX_form.html ), and the sequence alignments were completed using the ClustalX and MEGA5 software with the neighbour-joining method. The GhCYP82D1 and GhCYP82D2 promoter sequences were obtained through DNA walking in accordance with the Genome Walker Universal Kit User Manual (Clontech) using cv. YZ1 DNA as the PCR template. Plasmid construction and plant transformation The conserved region of the three SSN genes and 3′-UTR-specific regions of each gene were individually selected as the RNAi target and cloned into the RNAi vector pHellsgate 4 using the gateway system. Full-length SSN1 and SSN2 genes were amplified from the cv. YZ1 cDNA and cloned into pK2GW7,0 (Ghent University). The SSN1 and SSN2 promoters were fused with the GUS reporter gene in pGWB433 (Research Institute of Molecular Genetics, Shimane University, Matsue, Japan). The expression constructs were introduced into cv. YZ1 through the Agrobacterium tumefaciens strains LBA4404 or EHA105 (ref. 54 ). The TRV vectors were constructed, and the Agrobacterium tumefaciens (GV3101) were prepared for virus-induced gene silencing in accordance with a previous study [51] . The sequences used to construct TRV:GhLOX1 and TRV:GhLOX2 were amplified from the cv. YZ1 cDNA. The PCR fragments were digested with BamHI and KpnI and then ligated into the TRV:00 plasmid. The primer sequences are listed in Supplementary Table 2 . The vectors were used to transform A. tumefaciens through electroporation. The A. tumefaciens with TRV vectors were infiltrated into the 10-day-old YZ1 seedling cotyledons. The seedlings were then grown at 25 °C with a 16/8 h light/dark photoperiod in an incubator. Illumina sequencing analysis Total RNA was extracted using a plant total RNA kit (Sigma, St Louis, MO, USA) from 6-day-old Ri15 line and WT control seedling roots grown under identical conditions on a half-strength MS medium. RNA sequencing and data analysis were performed by the Beijing Genomics Institute (BGI, Shenzhen, China) using the Illumina Genome Analyzer. Briefly, the cDNA was digested with NlaIII and then ligated with the first adaptor containing the recognition site of MmeI, a type II endonuclease that cleaves at sites 21 bp from the recognition site. After digestion by MmeI, the transcripts were ligated with the second adaptor. Single-end sequencing mode was used and the read length was 49 bp. A sequence data set was constructed from cotton unigenes using NCBI ( http://www.ncbi.nlm.nih.gov/unigene/?term=txid3633 [Organism:exp]), which was used as the reference database. SOAPaligner/soap2 method was used to map reads and then the expression level of each gene was normalized to RPKM (reads per kb per million reads. The differential gene expression between WT and Ri15 was determined by taking the log2 ratio of RPKM. The Audic and Claverie method was used for normalization procedures and statistical data analysis [55] . FDR was used to determine the threshold of P value in multiple test and analysis. The RPKM>15 in any one sample and the absolute value of log2 ratio >1 based on the FDR<0.001 were used as the threshold to judge the significance of gene expression difference. Histochemical assay For GUS detection, fresh tissues were collected from the SSN1 promoter::GUS plants and SSN2 promoter::GUS plants, dipped into pre-chilled 80% (v/v) acetone for 30 min, infiltrated into a staining solution under a vacuum for 15 min and then moved to 37 °C for 6 h. The staining solution was composed of 0.9 g l −1 5-bromo-4-chloro-3-indolyl-b-glucuronic acid, 50 mM sodium phosphate buffer (pH 7.0), 20% (v/v) methanol and 100 mg l −1 chloromycetin. The samples were successively washed with 75% ethanol and then examined and photographed with a Nikon D40 camera (Japan). For H 2 O 2 detection, the stems without a lesion phenotype in SSN -RNAi and WT plants were sampled for H 2 O 2 measurements as described previously [56] . For DAB staining, SSN -RNAi plant cotyledons were incubated in 1 mg ml −1 pH 3.8 DAB-HCl (Sigma-Aldrich, USA) in the dark for 8 h. The cotyledons were then cleared by boiling in alcoholic lactophenol (95% ethanol:lactophenol, 2:1 v/v) for 20 min. The reddish colour of the cotyledons was used as evidence of H 2 O 2 and visualized using a Nikon D40 camera (Japan). For 2′,7′-DCFDA staining, the hypocotyls of each lines were excised from 9-day-old seedlings, which have no lesion phenotype on stems on media and cut into about 5-mm segments, then incubated for 30 min in the dark at 30 °C in 2′,7′-DCFDA diluted with phosphate buffer solution to 10 μM. The images were observed and recorded using an Olympus light microscope equipped with an Olympus U-PMTVC adapter and a Leica DC300F camera. For section observation, the hypocotyls of each lines were excised from 9-day-old seedlings, which have the weak lesion spot on stems on media and cut into 5–7 mm segments, and then were fixed in FAA solution (formaldehyde:acetic acid: 70% alcohol:water, 1:1:10:8) overnight at 4 °C. Samples were dehydrated in a progressive series of ethanol dilution, infiltrated in chloroform overnight at 37 °C and embedded in paraffin wax (melting point 56 °C). Sections (8 μm) were prepared using a rotary microtome (KD 2058, KEDEE, China) and stained with Safranin fast green. The sections were observed and photographed under a photomicroscope (DM2500, Leica, Wetzlar, Germany). More than 10 samples of each line were analysed above. Transmission electron microscopy scanning WT and transgenic seedling cotyledons were grown for 6 days under identical conditions, cut into 1 mm 2 pieces with a scalpel, prefixed in the fixing solution (2.5% glutaraldehyde adjusted to pH 7.4 with 0.1 M phosphate buffer and fixed in 2% OsO4 in the same buffer) and then cut into smaller pieces with scissors. Ultrathin sections were obtained using a Leica UC6 ultramicrotome (Leica, Germany) and stained with uranyl acetate then with lead citrate. The images were observed and recorded using a HITACHI H-7650 transmission electron microscope (Hitachi High-tech, Ibaraki-ken, Honshu, Japan) at 80 KV and a Gatan 832 CCD camera (Gatan, Pleasanton, CA). Quantitative real-time reverse transcription-PCR The total RNA was isolated as previously described [57] . Tissues were ground in a mortar with liquid nitrogen and ice-cold extraction buffer containing 1% β-mercaptoethanol was added and mixed completely by inverting the tube. The supernatant was purified by phenol and chloroform. The RNA was precipitated by isopropanol and sodium acetate (3 M) and then washed by 75% ethanol. Air-dried RNA was dissolved in diethylpyrocarbonate-treated water. The RNA was reverse transcribed to cDNA using the SuperScript III reverse transcriptase (Invitrogen). Quantitative real-time (qRT) PCR was performed using the ABI Prism 7000 system (Applied Biosystems, Foster City, CA, USA). For qRT-PCR analysis, at least 5–10 plants of every line or treatment were sampled for each independent biological replicate. Gene sequences were obtained from the public NCBI UniGene data bank. The primers are listed in Supplementary Table 2 . Four technical replicates or three biological replicates for each experiment were performed. Error bars represent the s.d. UBQ7 was amplified as a control. The expression value of all genes was normalized by referring to UBQ7 as ‘1’. Southern, northern and western blotting Genomic DNA was extracted from young leaves of transgenic cotton lines using the plant genomic DNA kit DP305 (Tiangen Biotech, Beijing). The NPTII gene was used as a probe for Southern blotting to detect transgene insertion. Total RNA from the leaves of 3-week-old seedlings was extracted as described above; a PR1 fragment was used as the probe for northern blot analysis in SSN -RNAi plants. Procedures for hybridization and washing the membrane were as previously reported [56] . The primer sequences are listed in Supplementary Table 2 . For western blotting, a specific amino acid sequence from the same region of SSN1 and SSN2 (residues 272–286 DHRKGGRWDENKKEK) was used as the antigen through commercial synthesis; the antibody was prepared by Neweast Bioscience (Wuhan, China). Anti-histone 3 (ab1791, Rabbit polyclonal to Histone H3—ChIP Grade, ABcam, San Francisco, CA) was used as an endogenous standard. Total protein was extracted from WT, SSN -RNAi and overexpressing seedlings using the extraction buffer. Protein concentrations were determined using the Bradford assay. Western blot experiments were performed as described previously [58] . The primary antibody was diluted at 1:5,000 for SSN probing or 1:10,000 for histone probing. A secondary anti-rabbit horseradish peroxidase labelled IgG was subsequently added. Signal of protein was detected using the Pierce Supersignal West Pico kit (Thermo Scientific, Rockford, IL). Transient expression and subcellular localization Full-length SSN1 cDNA without a stop codon was isolated using the primers forward, 5′-GGGGACAAGTTTGTACAAAAAAGCAGGCTTCATGGATCTTCTTGATTTCTCCACT-3′, and reverse, 5′-GGGGACCACTTTGTACAAGAAAGCTGGGTTGTTATAGAGCTCAGGAGCAAGGC-3′, carrying the attB adapter sites and recombined into the vector pMDC83 (ref. 59 ) by BP and LR recombination reactions (Gateway Technology); the resulting construct consisted of SSN1 fused to the green fluorescent protein N terminus controlled by the CaMV 35S promoter. An RFP fusion with the chaperone-binding protein BiP was used as an endoplasmic reticulum marker protein. The fusion constructs were introduced into Nicotiana benthamiana protoplasts isolated from seedling leaves by polyethylene glycol/calcium-mediated transformation [60] . Fluorescence microscopy was performed using a Leica TCS SP2 confocal spectral microscope (Leica, Heidelberg, Germany). Lipid analysis WT and transgenic plant cotyledons were quickly immersed in 3.0 ml 75 °C isopropanol with 0.01% butylated hydroxytoluene for 15 min. The mixture was vortexed after adding 1.5 ml chloroform and 0.6 ml water; it was then agitated (on shaking incubator) at room temperature for 1 h. The lipid extracts were transferred to glass screw-cap (Teflon-lined) tubes. Next, 4.0 ml chloroform/methanol (2:1) with 0.01% butylated hydroxytoluene was added before shaking for 30 min. The above procedure was repeated for all samples until the leaves of each sample became white. The process typically required approximately five extractions, including the isopropanol extraction. KCl (1 M, 1.0 ml) was added to the combined extract, the sample mixed by vortexing or shaking, then centrifuged to break up the phases and the upper phase was discarded. Water (2.0 ml) was added, vortexed or shaken, centrifuged and the upper phase was discarded. Extracted leaves were dried at 80 °C in an oven overnight for dry weight determination to four decimal places (0.0000, g). Samples were analysed by the KLRC (Kansas Lipidomics Research Center). The free fatty acids were analyzed in the (Applied Biosystems) API4000 triple quad mass spec using the negative MS1 scan mode. The source temperature was 100 °C, the desolvation temperature was 250 °C, 2.8 kV was applied to the electrospray capillary, the cone energy was 40 V and argon was used as the collision gas at 1.7 e −3 mBar as measured on the gauge in the collision cell line. Phytohormone and oxylipin quantitation For JA analysis, the samples (100–200 mg) were extracted twice with 80% cold methanol (v/v) overnight at 4 °C. To each sample was added 10 ng (±)-9,10-dihydro-JA (Olchemim) as an internal standard. The combined extract was evaporated to the aqueous phase with N 2 , dissolved in 0.4 ml methanol and then filtered using a syringe-facilitated filter (Nylon 66; Jin Teng Experiment Equipment Co., Tianjin, China). The samples were stored at −80 °C before the measurements. The JA levels were quantified using an HPLC-MS/MS system (AB SCIEX Triple Quad 5500 LC/MS/MS) with JA (Sigma) as the external standards. For JA-Ile and SA analysis, the JA-Ile and SA levels were quantified with JA-Ile and SA (Sigma) as the external standards. To estimate the oxylipins levels, the samples were obtained and extracted as described for phytohormone analysis. The supernatants were analysed using an HPLC-MS/MS system (AB SCIEX Triple Quad 5500 LC/MS/MS system) with 9- or 13-HPOD, 9- or 13-HPOT, 9- or 13-HOD, 9- or 13-HOT or 9- or 13-KOD (Cayman Chemical Co) as the external standard. Accession codes: cDNA sequences have been deposited in the NCBI GenBank database with the following accession codes: GhCYP82D1 (SSN1), KJ704109 ; cDNA of GhCYP82D2 (SSN2), KJ704110 ; cDNA of GhCYP82D3 (SSN3), KJ704111 . Raw RNA-seq data have been deposited in the Sequence Read Archive (SRA) under accession codes SRR1569164 . How to cite this article : Sun, L. et al. Cotton cytochrome P450 CYP82D regulates systemic cell death by modulating the octadecanoid pathway. Nat. Commun. 5:5372 doi: 10.1038/ncomms6372 (2014).